Reconstructing Austronesian population history in Island Southeast Asia Austronesian languages are spread across half the globe, from Easter Island to Madagascar. Evidence from linguistics and archaeology indicates that the ‘Austronesian expansion,’ which began 4,000–5,000 years ago, likely had roots in Taiwan, but the ancestry of present-day Austronesian-speaking populations remains controversial. Here, we analyse genome-wide data from 56 populations using new methods for tracing ancestral gene flow, focusing primarily on Island Southeast Asia. We show that all sampled Austronesian groups harbour ancestry that is more closely related to aboriginal Taiwanese than to any present-day mainland population. Surprisingly, western Island Southeast Asian populations have also inherited ancestry from a source nested within the variation of present-day populations speaking Austro-Asiatic languages, which have historically been nearly exclusive to the mainland. Thus, either there was once a substantial Austro-Asiatic presence in Island Southeast Asia, or Austronesian speakers migrated to and through the mainland, admixing there before continuing to western Indonesia. The history of the Austronesian (AN) expansion and of populations speaking AN languages has long been of interest. Patterns of lexical diversity within the AN language family point to Taiwan as the AN homeland [1] , [2] , as do elements of the archaeological record, for example, red-slipped pottery and Taiwanese-mined nephrite [3] , [4] , [5] . However, some authors have argued that the AN expansion was driven primarily by cultural diffusion rather than large-scale migration [6] , [7] , [8] , and other associated artifacts, such as cord-marked and circle-stamped pottery, likely derive instead from the mainland [9] , [10] . It is also unknown how the history of populations in western Island Southeast Asia (ISEA), which speak Western Malayo-Polynesian AN languages, differs from that of Central and Eastern Malayo-Polynesian speakers in eastern Indonesia and Oceania. Genetic data can be used to trace human migrations and interactions in a way that is complementary to the information provided by linguistics and archaeology. Some single-locus genetic studies have found affinities between Oceanian populations and aboriginal Taiwanese [11] , [12] , [13] , [14] , [15] , but others have proposed that present-day AN speakers do not have significant genetic inheritance from Taiwan [16] , [17] , [18] . Within Indonesia, several surveys have noted an east–west genetic divide, with western populations tracing a substantial proportion of their ancestry to a source that diverged from Taiwanese lineages 10,000–30,000 years ago (kya), which has been hypothesized to reflect a pre-Neolithic migration from Mainland Southeast Asia (MSEA) [19] , [20] , [21] , [22] . Genome-wide studies of AN-speaking populations, which in principle can provide greater resolution, have been interpreted as supporting both Taiwan-centered [23] , [24] and multiple-wave [21] models. However, such work has relied primarily on clustering methods and fitting bifurcating trees that do not model historical admixture events, even though it is well known that many AN-speaking populations are admixed [21] , [24] , [25] , [26] , [27] , [28] . Thus, these studies have not established firmly whether AN speakers have ancestry that is descended from Taiwan, MSEA or both. Here, we explore these questions by reconstructing the genome-wide ancestry of a diverse sample of AN-speaking populations, predominantly within ISEA. We apply novel methods for determining the phylogenetic placement of sources of gene flow in admixed populations and identify four major ancestry components, including one linked to Taiwan and a second Asian component from MSEA. Analysis of admixed populations To investigate the ancestry of AN-speaking populations at high resolution, we analysed a genome-wide data set of 31 AN-speaking and 25 other groups from the HUGO Pan-Asian SNP Consortium [25] and the CEPH-Human Genome Diversity Panel (HGDP) [29] . 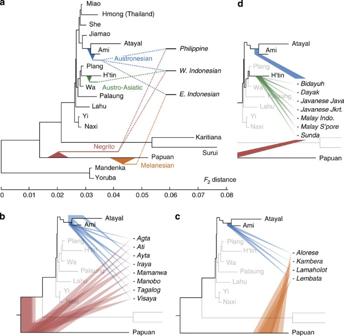Figure 1: Inferred sources of ancestry for selected admixed Austronesian-speaking populations. Shaded ranges represent 95% bootstrap confidence intervals for branching positions; seeSupplementary Tables 10 and 11for complete mixing branch distributions. The topology of the scaffold tree is shown using the full data set (slight variations are possible across bootstrap replicates). (a) Overview of the three best-fitting admixture models. (b–d) Detailed results for highest-confidence models of populations from (b) the Philippines, (c) eastern Indonesia and (d) western ISEA. Ind, the Austronesian and Negrito branch positions are fixed inMixMapperto equal those for Manobo. Batak Toba are omitted for display purposes, as 8% of replicates place their third ancestry component on a non-adjacent branch in the scaffold (Supplementary Table 11). Three other populations (Manggarai Ngada, Manggarai Rampasasa and Toraja) fall into an additional category of three-way admixed eastern Indonesians, while Oceanians (Fiji and Polynesia) are inferred to have similar ancestry to the populations inc, but their confidence intervals are not directly comparable because they have fewer SNPs available (seeFig. 2andSupplementary Tables 10 and 11). We used genotypes from 18,412 single-nucleotide polymorphisms (SNPs) that overlapped across all samples (see Methods, Supplementary Table 1 , and Supplementary Fig. 1 ). To confirm that our results are robust to the way SNPs were chosen, we repeated our primary analyses with data obtained by merging the Pan-Asia genotypes with HGDP samples typed on the Affymetrix Human Origins array [30] (see Methods and Supplementary Tables 2 and 3 ). For some tests requiring denser markers, we also used a smaller set of 10 AN-speaking groups first published in ref. 27 and typed at over 500,000 SNPs. We developed new methods to analyse the data, which we release here as the MixMapper 2.0 software. MixMapper is a tool for building phylogenetic models of population relationships that incorporate the possibility of admixture. Both the original version [31] and MixMapper 2.0 use allele frequency correlations to construct an unadmixed scaffold tree and then add admixed populations. The entire best-fitting model for each admixed population, including mixture proportions and the placement of the sources of ancestry on the scaffold, is inferred from the data, and uncertainty in parameter estimates is measured through bootstrap resampling (see Methods). MixMapper 2.0 substantially improves the three-way mixture fitting procedure of the original programme, as it implements a rigorous test to determine whether populations are best modelled via two- or three-way admixtures. It also allows for full optimization of the inferred mixture proportions (see Methods). A strength of MixMapper and related methods is that the underlying allele frequency correlation statistics, and hence the inferences about population relationships, are largely robust to the way that SNPs are chosen for analysis [30] , [31] , [32] . We selected a scaffold tree consisting of 18 populations that are approximately unadmixed relative to each other ( Fig. 1 ; Supplementary Tables 4 and 5 ): Ami and Atayal (aboriginal Taiwanese); Miao, She, Jiamao, Lahu, Wa, Yi and Naxi (Chinese); Hmong, Plang, H’tin and Palaung (from Thailand); Karitiana and Suruí (South Americans); Papuan (from New Guinea); and Mandenka and Yoruba (Africans). This set was designed to include a diverse geographical and linguistic sampling of Southeast Asia (in particular Thailand and southern China) along with outgroups from other continents, which are necessary for accurate mixture fitting [31] (see Methods). We have previously shown that MixMapper results are robust to the choice of scaffold populations [31] , and indeed our findings here were essentially unchanged when we repeated our analyses with an alternative, 15-population scaffold ( Supplementary Fig. 2 ; Supplementary Tables 6 and 7 ) and with 17 perturbed versions of the original scaffold ( Supplementary Tables 8 and 9 ). Using this scaffold tree, we obtained confident results for 25 AN-speaking populations (for geographical locations, see Fig. 2 ): eight from the Philippines, nine from eastern Indonesia and Oceania and eight from western ISEA. Several populations in our data set—Batak Karo, Ilocano, Malay, Malay Minangkabau, Mentawai and Temuan—were not as readily fit with MixMapper , which we hypothesize was due to the presence of additional ancestry components that we could not capture well in our modelling framework. Thus, we omit these populations from further analyses, although we note that their MixMapper results, while not as reliable, were still similar to those for the 25 groups discussed here. Figure 1: Inferred sources of ancestry for selected admixed Austronesian-speaking populations. Shaded ranges represent 95% bootstrap confidence intervals for branching positions; see Supplementary Tables 10 and 11 for complete mixing branch distributions. The topology of the scaffold tree is shown using the full data set (slight variations are possible across bootstrap replicates). ( a ) Overview of the three best-fitting admixture models. ( b – d ) Detailed results for highest-confidence models of populations from ( b ) the Philippines, ( c ) eastern Indonesia and ( d ) western ISEA. In d , the Austronesian and Negrito branch positions are fixed in MixMapper to equal those for Manobo. Batak Toba are omitted for display purposes, as 8% of replicates place their third ancestry component on a non-adjacent branch in the scaffold ( Supplementary Table 11 ). Three other populations (Manggarai Ngada, Manggarai Rampasasa and Toraja) fall into an additional category of three-way admixed eastern Indonesians, while Oceanians (Fiji and Polynesia) are inferred to have similar ancestry to the populations in c , but their confidence intervals are not directly comparable because they have fewer SNPs available (see Fig. 2 and Supplementary Tables 10 and 11 ). 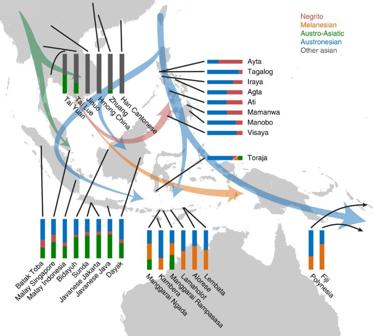Figure 2: Locations and best-fit mixture proportions for Austronesian-speaking and other populations, with possible directions of human migrations supported by our analyses. For Toraja, we could not distinguish between Negrito and Melanesian ancestry and show this component as red/orange. Full size image Figure 2: Locations and best-fit mixture proportions for Austronesian-speaking and other populations, with possible directions of human migrations supported by our analyses. For Toraja, we could not distinguish between Negrito and Melanesian ancestry and show this component as red/orange. Full size image All admixed AN-speaking populations fit best as combinations of two or three ancestry components out of a set of four: one closely related to Papuans (‘Melanesian’), one splitting deeply from the Papuan branch (‘Negrito’), one most closely related to aboriginal Taiwanese and one most closely related to H’tin ( Fig. 1 ). While the relative proportions varied substantially from group to group, the (independently inferred) positions of the ancestral mixing populations were highly consistent, leading us to assign them to these four discrete sources ( Fig. 1 ). A total of 14 populations were best modelled as two-way admixed ( Supplementary Table 10 ): all eight from the Philippines (with Taiwan-related and Negrito ancestry), four from eastern Indonesia (with Taiwan-related and Melanesian ancestry), and both from Oceania (Fiji and Polynesia, merged from ref. 27 ; also Taiwan-related and Melanesian). The remaining 11 populations, including all eight from western ISEA, fit best as three-way admixed ( Supplementary Table 11 ), with both Taiwan-related and H’tin-related ancestry ( Supplementary Table 12 ). Among the 25 groups, the Taiwan-related component was inferred to account for approximately 30–90% of ancestry, while for the 11 three-way admixed groups, the H’tin-related component was inferred to account for ~10–60%. By contrast, we found no Taiwan-related ancestry in admixed MSEA populations speaking non-AN languages ( Fig. 2 ; Supplementary Table 13 ). We note that our estimates of mixture proportions are robust to alternative histories involving multiple waves of admixture or continuous migration, since MixMapper is based on allele-sharing statistics that measure the probability of descent from each possible source of ancestry. Thus, continuous gene flow scenarios that preserve the same topology relating the admixed population to the scaffold tree will produce the same estimates of mixture proportions [30] , [31] . To obtain an independent estimate of how many sources of admixture are necessary to explain the observed relationships among populations from ISEA, we applied a formal test [33] , [34] that analyzes f 4 statistics among a set of admixed and outgroup populations to determine a lower bound on the total number of ancestry sources ( Supplementary Table 14 ). For the Philippines, we found that a maximal subset of six groups (Agta, Ati, Ayta, Ilocano, Iraya and Manobo) could be consistently modelled as derived from a single pair of mixing populations ( Supplementary Fig. 1A ). Likewise, the four eastern Indonesian groups (Alorese, Kambera, Lamaholot and Lembata) that were inferred to be two-way admixed by MixMapper could be modelled with two total ancestry sources according to the f 4 -based test ( Supplementary Fig. 1B ). However, adding the two Manggarai populations required a third source of ancestry, consistent with the H’tin-related ancestry inferred by MixMapper . In western ISEA, a large subset of six groups (Bidayuh, Dayak, Javanese Jakarta, Javanese Java, Mentawai and Sunda) was consistent with being derived from three ancestral mixing populations ( Supplementary Fig. 1C ), and moderately diverged subsets with as few as three populations (Bidayuh, Dayak and either Javanese or Sunda) still required three sources of ancestry. Larger subsets were always of greater complexity, indicating some additional, more localized gene flow, such as a likely influx of Indian ancestry in some populations [20] , [25] . However, the presence of the subsets that can be fit as mixtures of two or three sources increases our confidence that the MixMapper models are close to the true history. Finally, we used our recently developed ALDER software [35] to estimate the dates of admixture using linkage disequilibrium. For populations from the Philippines, eastern Indonesia, and Oceania from ref. 27 , we obtained dates of 30–65 generations ago assuming a single-pulse model of admixture (0.9–1.8 kya assuming 29 years per generation [36] ; Supplementary Fig. 3 ). These dates are considerably more recent than the initial AN expansion as documented through archaeology [2] , [3] , [4] , [5] , and thus they must reflect additional waves of interaction involving populations with different proportions of Asian ancestry after the initial AN settlement of the islands. We also applied ALDER to a merged set of populations from western ISEA and estimated that their admixture occurred 76±21 generations ago (2.2±0.6 kya; Supplementary Fig. 4 ). Again, this date implies the most recent possible time for the onset of population mixing and should not be interpreted as an estimate of the date of the earliest episodes of admixture [35] . Details of inferred ancestry components Our results indicate that there is a component of ancestry that is universal among and unique to AN speakers and that always accounts for at least a quarter of their genetic material. This component, moreover, is more closely related to aboriginal Taiwanese than to any population from the mainland. In theory, this ancestry could have been derived from a mainland source that was related to the ancestors of aboriginal Taiwanese but was either displaced by subsequent migrations (such as the expansion of Han Chinese) or whose descendants are not included in our data set. Given our dense sampling of East and Southeast Asian populations, this scenario seems unlikely, but we are unable to formally rule it out. We also considered the possibility that the direction of flow for this ‘Austronesian’ ancestry component could have been reversed, with an origin in Indonesia or the Philippines and a northward spread to Taiwan. Because of migrations, it is impossible to determine with certainty where ancestral populations lived based on present-day samples, but the fact that the aboriginal Taiwanese populations in our data set, Ami and Atayal, are unadmixed (to within the limits of our resolution), whereas the AN component appears in admixed form in all other AN-speaking populations from ISEA, can be most parsimoniously explained by a Taiwan-to-ISEA direction of gene flow. We verified that Ami and Atayal have no detectable signature of admixture both by the three-population test [30] , [37] ( Supplementary Table 5 ) and by testing them as putatively admixed in MixMapper with a scaffold tree made up of the other 16 original scaffold populations. In the latter analysis, we found that both Ami and Atayal returned best-fitting positions that indicated that they are properly modelled as unadmixed, adjacent to Jiamao ( Supplementary Table 15 ). On the other hand, all other AN-speaking populations, including those with no signal of admixture from the three-population test, continued to fit robustly as admixed on this reduced scaffold, with the AN component now closest to Jiamao, as expected ( Supplementary Table 15 ). Thus, the absence of admixture in Ami and Atayal allows us to conclude that they have a qualitatively different history from other AN-speaking populations in ISEA and that our inferred directionality of gene flow, with Taiwan as the source, is more parsimonious and a better fit to the data. The second and third ancestry components we infer for AN-speaking populations are Melanesian and Negrito. All admixed groups we tested contain at least one of these components, which we believe reflect admixture with indigenous populations in ISEA. The Melanesian component is closely related to Papuans and is found in the highest proportions among our study populations in easternmost Indonesia and in Fiji ( Fig. 2 ). The Negrito component, meanwhile, forms a deep clade with Papuans and is found in populations from the Philippines and western ISEA ( Fig. 2 ). We treat this ancestry as deriving from a single ancient source because it clusters phylogenetically across admixed populations, with the branching positions from the scaffold tree inferred to be very similar ( Fig. 1b ). We use the name ‘Negrito’ to describe this ancestry based on the fact that it occurs in the greatest proportion in Philippine Negrito populations. The Negrito ancestry in western ISEA could be a result of admixture with aboriginal people living on these islands or alternatively of prior admixture in the Philippines or on the mainland. We note that with MixMapper , we are unable to determine the precise branching position of this component in three-way admixed populations (see Methods), which would in principle shed light on this question. We are also unable to rule out a small proportion of Negrito ancestry in eastern Indonesia and Oceania—which might be plausible if AN speakers migrated from Taiwan through the Philippines first and admixed at that time with indigenous peoples—or a small proportion of Melanesian ancestry in the Philippines, but the large genetic drift separating the branching positions of the two components (Melanesian and Negrito) provides strong evidence that they reflect at least two ancestral sources ( Fig. 1 ). An unanticipated finding from our study is that populations in western ISEA, as well as a few in eastern Indonesia, also contain an unambiguous signal of an additional source of Asian ancestry, which is assigned with high confidence to an ancestral population splitting roughly two-fifths of the way down the H’tin branch in our scaffold tree ( Fig. 1d ). The H’tin speak a language belonging to the Austro-Asiatic (AA) family, which is hypothesized to have been the major language group in MSEA following the expansion of rice farming [5] . Later dispersals have resulted in substantial replacements of AA languages outside of Cambodia and Vietnam, but AA-speaking tribal groups are still present in areas where Tai, Hmong and Indo-European languages now predominate, extending as far west as India [5] . By contrast, no pockets of AA languages are found at all in present-day ISEA (with the exception of the Nicobar Islands in the Indian Ocean), which, in conjunction with the absence of clear archaeological evidence of previous settlement by agriculturalists who were not part of the AN cultural complex [10] , makes it unlikely that AA-speaking populations previously lived in the areas where we detect AA-related ancestry. To test the alternative explanation that the genetic evidence of AA-related ancestry in AN speakers might be an artifact of a back-migration from ISEA that contributed ancestry to the H’tin, we removed H’tin from our scaffold tree and repeated our analysis for three-way admixed populations. We found that the former H’tin-related ancestry component is now confidently inferred to form a clade with Plang (primarily) or Wa, both of which speak AA languages ( Supplementary Table 16 ). Similarly, when we also removed Plang, it formed a clade with Wa ( Supplementary Table 16 ). We also applied MixMapper to two admixed Negrito populations (Jehai and Kensiu) from peninsular Malaysia and found that their Asian ancestry component branches closest to H’tin, in almost exactly the same location as the H’tin-related component from ISEA. Since the Jehai and Kensiu speak AA languages, it is likely that the population contributing their Asian ancestry did as well, and AA-related populations may once have been more widespread in this region. We conclude that our signal indeed reflects gene flow from the mainland into ISEA from an ancestral population that is nested within the radiation of AA-speaking populations, and hence it is likely that this source population itself spoke an AA language. While a major AA contribution to western speakers of AN languages has not been proposed in the genetic literature, results from previous genetic studies are in fact consistent with these findings. A clustering analysis of the Pan-Asia SNP data [25] showed a component of ancestry in populations from (primarily western) ISEA that also appeared in AA speakers on the mainland, and a separate study of the same data also related western ISEA ancestry to mainland sources [21] . However, neither analysis concluded that these signals reflected an AA affinity. Our results are also compatible with published analyses of mtDNA and Y chromosomes, which have provided evidence of a component of ancestry in western but not eastern ISEA that is of Asian origin [20] , [21] , [22] . The O-M95 Y-chromosome haplogroup, in particular, is prevalent in western Indonesia [20] and was previously linked to AA-speaking populations [38] . A potential explanation for our detection of AA ancestry in ISEA is that a western stream of AN migrants encountered and mixed with AA speakers in Vietnam or peninsular Malaysia, and it was this mixed population that then settled in western Indonesia ( Fig. 2 ). This scenario is consistent with the AN mastery of seafaring technology and would be analogous to the spread of populations of mixed AN and Melanesian ancestry from Near Oceania into Polynesia [13] , [15] . Since we are unable to determine the date of initial AN–AA admixture, and genetic data from present-day populations do not provide direct information about where historical mixtures occurred, other scenarios are also conceivable; in particular, we cannot formally rule out a wider AA presence in ISEA before the AN expansion or a later diffusion of AA speakers into western ISEA. However, the absence of AA languages in Indonesia, together with our observation of both AA and AN ancestry in all surveyed western ISEA populations, suggests that the admixture took place before either group had widely settled in the region. We note that in its simplest form, the model of a single early admixture event would imply that populations today should have equal proportions of AN and AA ancestry, which is not the case for our sampled groups. However, these differences could have arisen through a number of straightforward demographic processes, including settlement of different islands by populations with different ancestry proportions, independent fluctuations within populations having heterogeneous ancestry soon after admixture, or continuous or multiple-wave gene flow over a number of generations. Overall, the uniformity of ancestry observed today, with the same components present in all of our sampled groups from western ISEA, points toward a shared mixture event rather than separate events for each population. These results show that the AN expansion was not solely a process of cultural diffusion but involved substantial human migrations. The primary movement, reflected today in the universally-present AN ancestry component, involved AN speakers from an ancestral population that is most closely related to present-day aboriginal Taiwanese. In western ISEA, we also find an Asian ancestry component that is unambiguously nested within the variation of present-day AA speakers, which makes it likely that the ancestral population itself spoke an AA language. Other suggestions of AN–AA interaction come from linguistics and archaeology [9] , as Bornean AN languages contain probable AA loan words [7] , and there is evidence that rice [3] , [6] , [7] , [10] and taro [7] cultivation, as well as domesticated pigs [39] , were introduced from the mainland. Interestingly, all languages spoken today in both eastern and western ISEA are part of the AN family, which raises the question of why AN languages were always retained by admixed populations. An important direction for future work is to increase the density of sampling of populations from Southeast Asia, with larger sample sizes and more SNPs, if possible in conjunction with ancient DNA [40] , to allow more detailed investigation of the dates and locations of the admixture events we have identified. Data set assembly For our primary analyses, we merged data from the HUGO Pan-Asian SNP Consortium [25] and the CEPH-HGDP [29] , yielding a set of 1,094 individuals from 56 populations typed at 18,412 overlapping SNPs. We excluded likely duplicate samples, twins and first-degree relatives from the Pan-Asia data (a total of 79 individuals) as identified in ref. 41 . We also removed 27 individuals identified as outliers by projecting each population onto principal components using EIGENSOFT [42] and deleting samples at least five standard deviations away from the population mean on any of the first three PCs. We also used 10 populations from ref. 27 , from a version of the published data set merged with HapMap3 (ref. 43 ) populations but not with Neanderthal and Denisova, for a total of 564,361 SNPs. We restricted to these populations when running ALDER and used all of the SNPs. We also merged these samples with our primary data set, leaving 7,668 SNPs, to estimate MixMapper parameters for Polynesia and Fiji. To test robustness to SNP ascertainment, we repeated our MixMapper analyses with a data set formed by merging the Pan-Asia data with HGDP samples typed on the Affymetrix Human Origins array [30] , replicating our primary data set on a different collection of 9,032 SNPs. Importantly, the Human Origins SNPs are chosen according to a very different strategy, having been selected based on their presence as heterozygous sites in sequenced genomes from diverse individuals. Full details for all analysed populations can be found in Supplementary Table 1 . Admixture inference with MixMapper The MixMapper software estimates admixture parameters using allele frequency moment statistics under a tree-based instantaneous admixture model [31] . The programme works in two phases. First, it constructs an (approximately) unadmixed scaffold tree via neighbour-joining on a subset of populations chosen by the user to have a specified level of geographic coverage with minimal evidence of admixture based on f -statistics [30] , [37] . The selection of populations for the scaffold is guided by running the three-population test [30] , [37] , which removes clearly admixed populations; by testing the additivity of possible subtrees from among the remaining populations (similar to the four-population test [30] , [37] ); and finally by comparing the fits of closely related candidate populations when modelled as admixed. After the scaffold is chosen, the software finds the best-fitting parameters for admixed populations by solving a system of moment equations in terms of the pairwise distance measure f 2 , which is the expected squared allele frequency difference between two populations. Specifically, the distance f 2 ( C , X ) between an admixed population C and each population X on the scaffold tree can be expressed as an algebraic combination of known branch lengths along with four unknown mixture parameters: the locations of the split points of the two ancestral mixing populations from the scaffold tree, the combined terminal branch length and the mixture fraction α . In this way, the entire tree topology can be determined automatically, even for large numbers of populations. Finally, MixMapper uses a nonparametric bootstrap [44] to determine confidence intervals for the parameter estimates, dividing the SNPs into 50 blocks and resampling the blocks at random with replacement for each of the 500 replicates. We note that the bootstrap is applied over the entire fitting procedure [44] , including the application of neighbour-joining to build the scaffold, so that uncertainty in the scaffold topology is accounted for in the final confidence intervals. For our analyses here, we developed new inference algorithms, released in the MixMapper 2.0 software, which extend the original MixMapper three-way mixture-fitting procedure, whereby one ancestral mixing population is taken to be related to a population already fit by the programme as admixed. First, MixMapper 2.0 implements a method to determine the best fit among alternative admixture models—namely, fitting a test population C either as two-way admixed or as three-way admixed with one ancestor related to a fixed admixed population A (for our applications, either Manobo or Alorese)—by comparing the norm of the vector of residual errors for all pairwise distances f 2 ( C , X ), where X ranges over the scaffold populations. Importantly, the two models have the same number of degrees of freedom, with four parameters being optimized in each case. Also, the comparison is restricted to those populations X on the initial scaffold, that is, we do not include f 2 ( C , A ) in the vector of residuals for the three-way model. Thus, our procedure is conceptually equivalent to augmenting the scaffold by adding A (via the standard MixMapper admixture model) and then finding the best-fitting placement for C . Second, for populations that are better fit as three-way admixed, MixMapper 2.0 implements improved estimation of their proportions of ancestry from all the three components by re-optimizing this same set of equations but now allowing all of the mixture fractions to vary (as well as the terminal branch lengths for the admixtures, since these depend on the mixture fractions [31] ). To prevent overfitting, we fix the branching positions of each ancestry component as determined from the initial fit (independently for each bootstrap replicate). How to cite this article : Lipson, M. et al. Reconstructing Austronesian population history in Island Southeast Asia. Nat. Commun . 5:4689 doi: 10.1038/5689 (2014).